Ultrasensitive and label-free molecular-level detection enabled by light phase control in magnetoplasmonic nanoantennas Systems allowing label-free molecular detection are expected to have enormous impact on biochemical sciences. Research focuses on materials and technologies based on exploiting localized surface plasmon resonances in metallic nanostructures. The reason for this focused attention is their suitability for single-molecule sensing, arising from intrinsically nanoscopic sensing volume and the high sensitivity to the local environment. Here we propose an alternative route, which enables radically improved sensitivity compared with recently reported plasmon-based sensors. Such high sensitivity is achieved by exploiting the control of the phase of light in magnetoplasmonic nanoantennas. We demonstrate a manifold improvement of refractometric sensing figure-of-merit. Most remarkably, we show a raw surface sensitivity (that is, without applying fitting procedures) of two orders of magnitude higher than the current values reported for nanoplasmonic sensors. Such sensitivity corresponds to a mass of ~0.8 ag per nanoantenna of polyamide-6.6 ( n =1.51), which is representative for a large variety of polymers, peptides and proteins. The most prominent routes for high-sensitivity and label-free detection in a compact device setting presently rely on localized surface plasmon resonance (LPR)-based technologies. The greatly enhanced electromagnetic fields at the surface of a resonant plasmonic nanostructure [1] , [2] allow for probing minute changes in the surrounding environment. Owing to the evanescent nature of the fields, the sensing volume of plasmonic nanostructures is only marginally larger than the structures themselves, making them ideal probes for localized changes in a medium. For these reasons, the utilization of LPRs for label-free molecular detection is under very active investigation for biochemical and biomedical applications [3] , [4] , [5] , [6] , [7] , [8] , [9] , [10] , [11] , [12] . They feature optical interrogation schemes, small footprint, high sensitivity of refractometric detection, potentially down to a single-molecule level because of the electromagnetic field enhancement at the nanoscale [3] , [4] , and easy integration with a wide range of fluidic systems for analyte delivery. To quantify the sensing performance of a LPR-based sensor, the bulk refractive index sensitivity S RI =Δ λ */Δ n is often considered, where Δ λ * is the shift of the LPR peak position λ * in nanometres measured in the extinction spectra over the change in the environment refractive index Δ n . For detection at the molecular level, sensitivity to local variation of the index of refraction is most relevant. In this case sensor performances are quantified in terms of surface sensitivity S Surf =Δ λ */Δ t at a given refractive index n , where t is the thickness of an assembled thin layer of the material with refractive index n being sensed on top of the active surface. Since the final accuracy of the peak tracking depends both on the magnitude of the peak shift and on the resonance line-width, the most crucial performance-defining parameter is the figure-of-merit (FoM), obtained by dividing either S RI or S Surf by the full width at half maximum (FWHM) of the resonance. Current LPR-based sensors have a surface FoM lower or at most comparable to that of propagating surface plasmon resonance (SPR)-based sensors [13] , [14] , [15] , which are the core and reference systems for label-free optical detection. However, SPR-based sensors are not an alternative for single-molecule level detection because of the lack of local sensitivity to the index of refraction. Therefore, tremendous research efforts aimed at improving the FoM of LPR-based sensors have been conducted [9] , [10] , [12] , [16] , [17] , [18] . Here we unveil a sensing modality that utilizes the unique optical properties of nanostructured magnetoplasmonic nanoantennas to combine and enhance all mentioned features of plasmonic sensing. Most importantly, we demonstrate that our approach delivers a manifold improvement of surface sensitivity and orders of magnitude higher surface FoM with respect to recent values reported for plasmonic-based detectors, including SPR-based sensors [14] , [15] , [18] . The proposed approach relies on magnetoplasmonic ferromagnetic (FM) nanoantennas deposited on a transparent substrate. FM nanoantennas are known to support LPRs [19] and, once activated by an external magnetic field, they acquire an intrinsic magneto-optical (MO) activity. The key point is the selection of the FM material and nanoantennas’ design in order to produce exact phase compensation in the electric field components of the otherwise elliptically polarized transmitted light at a specific wavelength λ ε . Under this condition, a vanishing ellipticity ε ( ε null-point, that is, full linear polarization) is produced at λ ε . Our underlying strategy relies on the fact that light polarization changes can be measured precisely especially near null conditions. The determination of λ ε provides a phase-sensitive identification of the nanoantennas’ LPR position and enables tracking of the spectral shift caused by local refractive index variations with unprecedented precision. Theoretical background In ferromagnetic bulk materials and continuous films, the MO activity is governed by the spin–orbit interaction, which is a property intrinsic to a given material. Conversely, the MO response of a magnetic nanoantenna is governed also by LPRs [19] , [20] , [21] , [22] , [23] , [24] . As depicted in Fig. 1 , light interacting with a magnetic field-activated FM nanoantenna excites two coupled LPRs, one directly driven by the electric field of the incident light and the second induced orthogonally by the inherent MO activity. Desired light polarization behaviour in transmission (and/or reflection) is achievable by tuning the relative phase of these two excited LPRs by designing the nanostructures. In detail, is the LPR polarized perpendicular to the driving electric field and light propagation direction that is governing the MO response of the nanoantenna. This fundamental physical effect can be visualized as follows: the incident electric field E x 0 induces an electric dipole along the x axis described as p x = α xx E x 0 , where α xx is the diagonal element of the polarizability tensor. The corresponding oscillation of the conduction electrons along the x axis is spin–orbit coupled with the magnetization M within the nanoantenna, which is aligned along the z axis by the applied magnetic field in the experimental geometry adopted here. This coupling induces an additional oscillation motion of conduction electrons, that is, a second electric dipole p y , along the in-plane transverse y axis direction. In general, the expression for the spin–orbit induced transverse dipole can be written conveniently in terms of the off-diagonal polarizability tensor elements α ij = ε ij α ii α jj /( ε 0 − ε m ) 2 , where ε ij and ε 0 , are the off-diagonal and diagonal elements of the dielectric tensor of the given constituent material, and ε m is the dielectric constant of the embedding medium. This expression shows that the off-diagonal elements of the polarizability tensor are proportional to the product between the diagonal components of the tensor along the two mixed directions. In the present case, the spin–orbit transversally induced dipole is given by p x = α yx E x 0 =[ ε yx α yy α xx /( ε 0 − ε m ) 2 ] E x 0 (considering the circular shape of our nanoantennas, α yy = α xx , that is, the two LPRs resonate at the same wavelength, and the expression above can be simplified to p x = α yx E x 0 =[ ε yx α 2 xx /( ε 0 − ε m ) 2 ] E x 0 ). 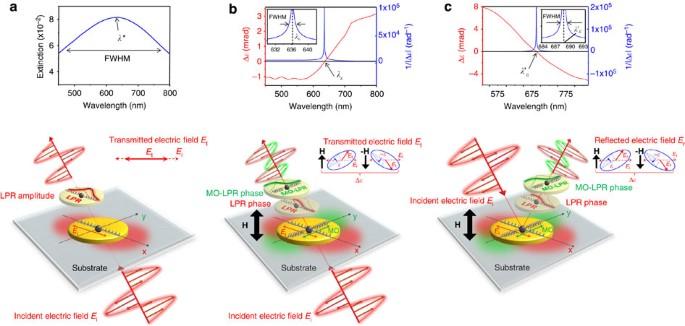Figure 1: LPR phase sensitivity in the transmitted light polarization. (a) When an incident light beam hits a ferromagnetic nanoantenna, the conduction electrons inside the nanostructure oscillate driven by the electric fieldEi. TheseEi-driven oscillations can be modelled as a damped spring-mass harmonic oscillator. A LPR is induced at a specific photon wavelengthλ*, yielding a peak in the extinction spectrum (I0−It)/I0=1−(Et/Ei)2, displayed in the top panel. (b) If the nanoantenna is magnetized perpendicularly to the surface plane, a MO-activity is turned on inducing a second MO-coupled LPR (MO-LPR) orthogonal to that directly driven byEi. In a circular nanoantenna the MO-LPR resonates at the sameλ*. The simultaneous excitation of LPR and MO-LPR induces an elliptical polarizationεof the transmitted fieldEt(refs20,21). The null conditionε=0 is generated at a desiredλε(in generalλε≠λ*) simply through engineering of the size of the circular nanoantenna21,34,35. Measurement ofλεprovides a precise phase-sensitive detection of the LPR position. The top panel displays typical Δεspectrum (red-line), as well as the 1/|Δε|spectrum (blue-line) and its resonance atλε. The close-up view of the 1/|Δε|spectrum aroundλεshown in the inset features a very narrow FWHM (~1.7 nm). (c) Similarly to the case described inb, the concerted action of the simultaneously excitated LPR and MO-LPR can be exploited to actively manipulate the reflected light’s polarization inducing the conditionε=0 at a desiredλ'ε. In general,λ'ε≠λεsince in this case also the additional phase introduced by the substrate reflectivity contributes to the polarization of the reflected fieldEr. As in transmission geometry, the detection ofλ'εprovides precise phase-sensitive detection of the LPR position. The top panel displays typical Δεspectrum (red line), as well as the 1/|Δε|spectrum (blue line) and its resonance atλ'ε. The close-up view of the 1/|Δε|spectrum aroundλ'εshown in the inset features a very narrow FWHM (<1.7 nm). Both in transmission and reflection, the sensitivity increases further by measuring the magnetic field-induced variation Δεasεreverses its sign upon invertingH(seeSupplementary Fig. 2). Figure 1: LPR phase sensitivity in the transmitted light polarization. ( a ) When an incident light beam hits a ferromagnetic nanoantenna, the conduction electrons inside the nanostructure oscillate driven by the electric field E i . These E i -driven oscillations can be modelled as a damped spring-mass harmonic oscillator. A LPR is induced at a specific photon wavelength λ* , yielding a peak in the extinction spectrum ( I 0 − I t )/ I 0 =1 − ( E t / E i ) 2 , displayed in the top panel. ( b ) If the nanoantenna is magnetized perpendicularly to the surface plane, a MO-activity is turned on inducing a second MO-coupled LPR (MO-LPR) orthogonal to that directly driven by E i . In a circular nanoantenna the MO-LPR resonates at the same λ* . The simultaneous excitation of LPR and MO-LPR induces an elliptical polarization ε of the transmitted field E t (refs 20 , 21 ). The null condition ε =0 is generated at a desired λ ε (in general λ ε ≠ λ* ) simply through engineering of the size of the circular nanoantenna [21] , [34] , [35] . Measurement of λ ε provides a precise phase-sensitive detection of the LPR position. The top panel displays typical Δ ε spectrum (red-line), as well as the 1/|Δ ε| spectrum (blue-line) and its resonance at λ ε . The close-up view of the 1/|Δ ε| spectrum around λ ε shown in the inset features a very narrow FWHM (~1.7 nm). ( c ) Similarly to the case described in b , the concerted action of the simultaneously excitated LPR and MO-LPR can be exploited to actively manipulate the reflected light’s polarization inducing the condition ε =0 at a desired λ' ε . In general, λ' ε ≠ λ ε since in this case also the additional phase introduced by the substrate reflectivity contributes to the polarization of the reflected field E r . As in transmission geometry, the detection of λ' ε provides precise phase-sensitive detection of the LPR position. The top panel displays typical Δ ε spectrum (red line), as well as the 1/|Δ ε| spectrum (blue line) and its resonance at λ' ε . The close-up view of the 1/|Δ ε| spectrum around λ' ε shown in the inset features a very narrow FWHM (<1.7 nm). Both in transmission and reflection, the sensitivity increases further by measuring the magnetic field-induced variation Δ ε as ε reverses its sign upon inverting H (see Supplementary Fig. 2 ). Full size image Notably, the transversally induced electric dipole p y is of second order in terms of polarizability as it depends on the product of two polarizabilites, α xx and α yy , while the directly induced dipole p x depends only on α xx . This difference is crucial for the present application and can be understood considering that the transverse oscillation is not driven directly by E x 0 but by the induced dipole p x with the mediation of the spin–orbit coupling. The polarization state of the far-field radiated in the z direction, either transmitted or reflected (Faraday or Kerr geometry), can be represented by the ratio of these two in-plane and mutually orthogonal oscillating electric dipoles, namely by the complex MO polarization angle Θ =p y / p x = ε yx α xx /( ε 0 − ε m ) 2 . This expression reveals that the polarization of the transmitted and reflected light is governed by both the intrinsic properties of the constituent material [ α M = ε yx /( ε 0 − ε m ) 2 ] and by the in-plane LPR in the nanoantenna ( α yy , which coincides with α xx for circular nanoantennas). In detail, the transmitted and reflected light will have an elliptical polarization described through measurable rotation and ellipticity angles given by θ =Re(Θ) and ε =Im(Θ), respectively. Physically, both θ and ε at any light wavelength are determined by the relative phase ΔΦ of the two scattering electric dipoles p x and p y , since the complex MO angle Θ ∝ e i ΔΦ , where ΔΦ =Φ [ α M ]+Φ [ α yy ]. For a given constituent material Φ [ α M ] is fixed. A null condition ε =0 (ΔΦ=0, π, 2π…) can be generated at a desired λ ε simply through engineering of the size of the circular nanoantenna, which controls both the spectral position and phase Φ [ α yy ] of the LPR [21] . As a result, measuring λ ε provides a precise and phase-sensitive detection of any shift of the LPR position ( λ ε and λ * are not bound to be identical) induced by modifications of the dielectric properties of the near-field region local environment. Bulk refractive index sensitivity The magnetoplasmonic nanostructures investigated here are bottom-up, short-range-ordered nickel (Ni) cylindrical nanoantennas on glass ( Fig. 2a ) [25] . For determining S RI , we measured the extinction spectra by immersing the samples in solutions with different indices of refraction n ( Fig. 2b and Supplementary Fig. 1 ). The observed shift of λ * leads to S RI of 180 and 230 nm per refraction index unit (nm RIU −1 ) for 30-nm-thick Ni nanoantennas with diameters of 100 and 160 nm, respectively (upper panels of Fig. 2b and Supplementary Fig. 1 ). In parallel, we determined the null-point wavelength λ ε by measuring the spectral dependence of the polarization ellipticity variation Δ ε of the transmitted light, induced by applying and reversing the MO activation field H (Methods and Supplementary Fig. 2 ). The wavelength λ ε is more precisely visualized by plotting the quantity 1/|Δ ε |, which resonates at λ ε , as shown in the top panels of Figs 1b-1c . Plotting the data in this manner makes it much easier to visualize the enormous gain in precision (limit of detection) and sensitivity of our approach. In addition, and for the sake of direct comparison with the FoM, which is conventionally utilized for defining the performances of a plasmonic detector, the plot of 1/|Δ ε | provides the most sensible way to perform this comparison. We make it clear that comparison between sensitivity (both bulk and surface) and limit of detection performances of our approach with respect to plasmonic-based sensors are instead derived from direct measurements of Δ ε spectra and the precision (noise level) with which λ ε is determined from such measurements. 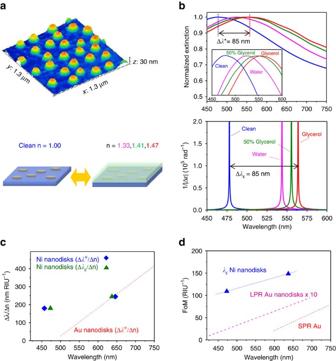Figure 2: Refractive index sensitivity of Ni magnetoplasmonic nanoantennas. (a) 3D AFM profile of Ni magnetoplasmonic nanoantennas on glass, with lateral dimensions of 103±5 nm (diameter) and 30±0.5 nm (thickness). (b; Top panel) extinction spectra of Ni cylindrical nanoantennas for different values of the embedding refractive index (cleann=1, watern=1.33, 50% Vol. glyceroln=1.41 and glyceroln=1.47; the inset shows a zoom of the resonance peaks in the spectral region 450–600 nm; bottom panel) plot of the inverse of transmitted light ellipticity variation 1/|Δε| for the same values of the embedding refractive index as above. (c) Comparison between the bulk sensitivities of Au26(Δλ*/Δn; red-dashed line) and Ni (both Δλ*/Δnand Δλε/Δn; blue and green markers, respectively) cylindrical nanoantennas on glass. (d) Comparison between the bulk figure-of-merit of Au26[(Δλ*/Δn)/FWHM] (purple dashed line) and Ni [(Δλε/Δn)/FWHM] (blue markers are experimental data, blue dotted line is a guide for eyes) cylindrical nanoantennas, and Au surface plasmon resonance14(red dashed line), in the spectral range 420–750 nm. Figure 2: Refractive index sensitivity of Ni magnetoplasmonic nanoantennas. ( a ) 3D AFM profile of Ni magnetoplasmonic nanoantennas on glass, with lateral dimensions of 103±5 nm (diameter) and 30±0.5 nm (thickness). ( b ; Top panel) extinction spectra of Ni cylindrical nanoantennas for different values of the embedding refractive index (clean n =1, water n =1.33, 50% Vol. glycerol n =1.41 and glycerol n =1.47; the inset shows a zoom of the resonance peaks in the spectral region 450–600 nm; bottom panel) plot of the inverse of transmitted light ellipticity variation 1/|Δ ε | for the same values of the embedding refractive index as above. ( c ) Comparison between the bulk sensitivities of Au [26] (Δ λ */Δ n ; red-dashed line) and Ni (both Δ λ */Δ n and Δ λ ε /Δ n ; blue and green markers, respectively) cylindrical nanoantennas on glass. ( d ) Comparison between the bulk figure-of-merit of Au [26] [(Δ λ */Δ n )/FWHM] (purple dashed line) and Ni [(Δ λ ε /Δ n )/FWHM] (blue markers are experimental data, blue dotted line is a guide for eyes) cylindrical nanoantennas, and Au surface plasmon resonance [14] (red dashed line), in the spectral range 420–750 nm. Full size image The spectra of 1/|Δ ε | for the two studied samples and for different values of n are shown in the lower panels of Fig. 2b and Supplementary Fig. 1 . We observe that λ ε undergoes a shift equal to that of λ *, confirming the S RI values determined above. It is clear that monitoring λ ε instead of the extinction peak λ * enables tracking of the resonance shift with an exceptionally higher precision. In principle, our approach is characterized by a virtually unlimited value of the FoM since 1/|Δ ε | is diverging at the resonant wavelength λ ε . Practically, however, we can estimate a FWHM by accounting for experimental errors. Although polarization parameters can be determined with submicro-radiant resolution (down to 10 nrad), here we assume an experimental resolution of 5 micro-radians in the determination of Δ ε , which is easily achievable without the utilization of advanced tools and/or fitting procedures, and consequently truncate the 1/|Δ ε | spectra at 2 × 10 5 rad −1 (see the insets of the top panels of Figs 1b-1c ). We obtain a FWHM ranging from 1.5 to 1.8 nm for the resonance of the 1/|Δ ε | spectra ( Fig. 2b and Supplementary Fig. 2 ). Taking the average FWHM of ~1.7 nm means a FoM of more than 100 RIU −1 and approaching 150 RIU −1 for Ni nanoantennas with diameters of 100 and 160 nm, respectively. Such large FoM values greatly exceed even those for SPR in the same spectral range, which are often considered as theoretical limit references [10] . Figure 2c,d shows a comparison of the sensitivities of Au and Ni cylindrical nanoantennas on glass as well as their FoM, including that of SPR-based sensors. The outstanding sensing performance of our magnetoplasmonic nanoantennas is better appreciated if compared directly with recently developed nanoplasmonic sensors. Improvements in FoM have been achieved by boosting the S RI and/or reducing the FWHM of the LPR. S RI enhancement has been realized by lifting metal nanostructures above substrates with dielectric pillars in order to expose more efficiently the surrounding environment to the LPR-enhanced electric field [26] . More efforts have been devoted to a reduction of the FWHM of LPRs caused by inherent losses in metallic nanostructures. The most effective approach relies on resonant coupling of LPRs with modes that possess a smaller FWHM. Such modes could, for example, be SPRs in an optically coupled thin metallic continuous layer [16] , diffractive coupling among the nanostructures arranged in periodic arrays [15] , and coherent coupling of different localized plasmon modes in nanostructures with complex shapes [9] , [17] . FoM values towards ~60 have been reported upon resonant coupling of LPRs and SPRs [16] . More recently, a FoM value of up to 108 has been reported from periodic arrays of gold ‘nano-mushrooms’ that combine the two aforementioned approaches [10] . It is worth noting that all pathways towards enhancement of the FoM rely on a substantial increase in the complexity of the plasmonic nanostructures and arrangements design. In addition, the performance boost applies to a specific and narrow wavelength range where resonant coupling occurs. By exploiting the built-in phase sensitivity of the individual magnetoplasmonic nanoantennas, we circumvent the limitation due to their inherent losses, while keeping the nanostructuring process extremely simple and maintaining the outstanding performance over a broad spectral range. Surface sensitivity Applications to molecular detection rely on high sensitivity and FoM to the local variation of the index of refraction n . A reliable and precise assessment of the detection performance is an experimental challenge, as control of Δ n on the molecular level is needed. The method of choice is the controlled deposition of extremely thin and removable films using molecular layer deposition (MLD), an organic variant of atomic layer deposition [27] , [28] . The cyclic and self-terminating growth mechanisms of this method allow molecular-scale control of the polymer film growth and surface-dependent nucleation characteristics can be used for area-selective growth through matching of substrate and precursor chemistries. More importantly, MLD deposits polymer films from vapourized pure molecular fragments avoiding potentially negative impact of solvents (see also Methods). For our experiments we used MLD of polyamide 6.6 (PA-6.6) with n =1.51 (ref. 28 ). This polymer was chosen for convenience as the MLD process is well established and also, being a polyamide, it is representative for a large variety of polymers, peptides and proteins. In a first experiment, PA-6.6 was deposited 20 cycles at a time. The film thickness was measured by atomic force microscopy (AFM). The corresponding change of the local index of refraction was monitored by tracking λ ε . Since the surface was modified only locally, we conducted polarization measurements also in reflection geometry as an alternative way to track λ ε (see Fig. 1c ). The experimental spectra and the resulting shift of λ ε are shown in Fig. 3a,b . AFM images and their quantitative analysis show that PA-6.6 nucleated selectively on the Ni nanodisks and linearly grew up to ~100 cycles ( Fig. 3c,d ). Combining the two plots in Fig. 3b,d , we find S Surf values of ~3 and ~5.3 in transmission and reflection geometry, respectively. The remarkable enhancement by a factor 1.7 of the S Surf in reflection geometry, confirmed also by calculations, is a consequence of a larger shift of λ ε caused by the additional phase contribution of uncovered substrate reflectivity (details in Supplementary Fig. 3 ). Such S Surf value of ~5.3 is 3.5 times the surface sensitivity reported for Au-based SPR detectors in the same spectral region for the same refractive index [13] . Even more remarkable is the surface FoM ( S Surf /FWHM) of our magnetoplasmonic nanoantennas approach, whose value slightly larger than three is two orders of magnitude higher than the best surface FoM values achieved with plasmonic systems [14] . 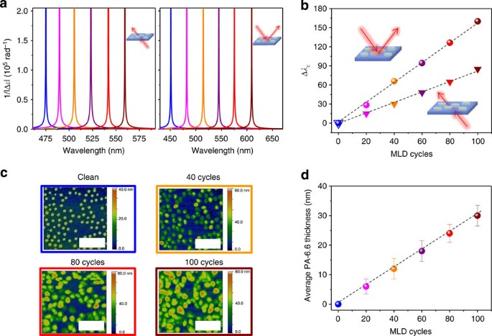Figure 3: Surface sensitivity assessment combining polarimetry and AFM measurements. (a) Plot of the inverse of the transmitted (left panel) and reflected (right panel) light ellipticity 1/|Δε| spectra as a function of MLD cycles (at steps of 20 cycles). (b) 1/|Δε| resonance wavelengthλεas a function of the MLD cycles for the two measurement geometries. In both cases, a linear dependence ofλεversus number of MLD cycles is observed (the black dashed lines are guide for eyes). The shift ofλεsaturates for a number of MLD cycles equal to 120, corresponding to a PA-6.6 thickness of ~35 nm, as shown inSupplementary Fig. 7for transmission geometry case. Such PA-6.6 thickness agrees well with the near-field spatial extension (seeSupplementary Fig. 4). (c) AFM images taken from the same sample region (total area imaged 2.7 × 2.7 μm2) after different numbers of MLD cycles. The AFM images show that PA-6.6 grows only on top of the nanoantennas. The colours of the frames refer to the corresponding coloured polarimetry (b) and thickness (d) data points. The length of the white scale bars in the images corresponds to 1 μm. (d) PA-6.6 average thickness as function of the MLD cycles after AFM topography image analysis. Surface sensitivities (spectral variation ofλεdivided by the average nylon thickness) of ~3 (transmission) and ~5.3 (reflection) are found combining plots (b,d). The error bars indicate the s.d. from the average thicknesses measured analysing the AFM images. Figure 3: Surface sensitivity assessment combining polarimetry and AFM measurements. ( a ) Plot of the inverse of the transmitted (left panel) and reflected (right panel) light ellipticity 1/|Δ ε | spectra as a function of MLD cycles (at steps of 20 cycles). ( b ) 1/|Δ ε | resonance wavelength λ ε as a function of the MLD cycles for the two measurement geometries. In both cases, a linear dependence of λ ε versus number of MLD cycles is observed (the black dashed lines are guide for eyes). The shift of λ ε saturates for a number of MLD cycles equal to 120, corresponding to a PA-6.6 thickness of ~35 nm, as shown in Supplementary Fig. 7 for transmission geometry case. Such PA-6.6 thickness agrees well with the near-field spatial extension (see Supplementary Fig. 4 ). ( c ) AFM images taken from the same sample region (total area imaged 2.7 × 2.7 μm 2 ) after different numbers of MLD cycles. The AFM images show that PA-6.6 grows only on top of the nanoantennas. The colours of the frames refer to the corresponding coloured polarimetry ( b ) and thickness ( d ) data points. The length of the white scale bars in the images corresponds to 1 μm. ( d ) PA-6.6 average thickness as function of the MLD cycles after AFM topography image analysis. Surface sensitivities (spectral variation of λ ε divided by the average nylon thickness) of ~3 (transmission) and ~5.3 (reflection) are found combining plots ( b , d ). The error bars indicate the s.d. from the average thicknesses measured analysing the AFM images. Full size image In order to demonstrate that very small quantities of material can be detected, PA-6.6 deposition, polarization ellipticity measurements and AFM characterization were performed sequentially for the very first cycles of MLD. 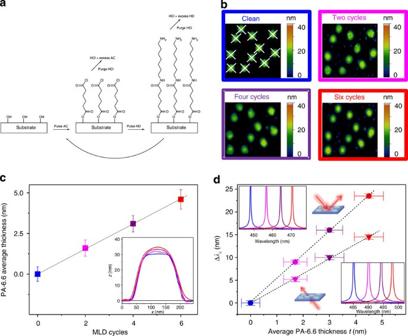Figure 4: Surface sensitivity in the first few cycles of PA-6.6 MLD. (a) Schematic of one cycle of the MLD process for PA-6.6. A substrate with –OH surface groups is exposed to a pulse of AC. The AC reacts with these –OH groups creating the by-product HCl, which is purged away along with any unreacted AC. Next, a pulse of HD is introduced to the reaction chamber and reacts with the available –Cl groups. Again, the by-product is HCl, which is purged away along with any unreacted HD. This process is repeated until the desired thickness is achieved. Nominally, the process has a growth rate of ~0.8 nm per cycle29. (b) AFM images taken from the same sample region (total area imaged 1.2 × 1.2 μm2) before and after PA-6.6 MLD. The colours of the frames refer to the corresponding coloured thickness (c) and polarimetry (d) data points. (c) PA-6.6 average thickness as function of the MLD cycles after AFM topography image analysis. The error bars indicate the s.d. from the average thicknesses shown in the inset, which shows the line profiles of all the disks included in the images inb. The line profiles are taken along two orthogonal directions, which are shown as white dashed lines only in the AFM image of the clean sample inb. (d) Plot of the inverse of transmitted and reflected light ellipticityλεas a function of MLD cycles (black dashed lines are guide for eyes). Surface sensitivities of ~3.1 (transmission) and ~5.4 (reflection) are found combining plots (c,d), in excellent agreement with the results presented inFig. 3. The horizontal error bars indicate the s.d. from the average thicknesses shown in the inset in (c). The vertical error bars indicate the experimental error in the magneto-optical measurements. The insets show the corresponding 1/|Δε| spectra for the two measurement geometries (reflection—top-left inset and transmission—bottom-right inset). Figure 4 shows that already after two MLD cycles an average increase in t of ~1.6 nm is determined by AFM. The resulting Δ λ ε for the two measurement geometries confirm the surface sensitivities obtained in the previous experiment. On the basis of our very conservative error bar estimate in the measurement of Δ ε , we can detect λ ε with ~0.5 nm precision without the application of any fitting procedure (raw limit of detection). Figure 4: Surface sensitivity in the first few cycles of PA-6.6 MLD. ( a ) Schematic of one cycle of the MLD process for PA-6.6. A substrate with –OH surface groups is exposed to a pulse of AC. The AC reacts with these –OH groups creating the by-product HCl, which is purged away along with any unreacted AC. Next, a pulse of HD is introduced to the reaction chamber and reacts with the available –Cl groups. Again, the by-product is HCl, which is purged away along with any unreacted HD. This process is repeated until the desired thickness is achieved. Nominally, the process has a growth rate of ~0.8 nm per cycle [29] . ( b ) AFM images taken from the same sample region (total area imaged 1.2 × 1.2 μm 2 ) before and after PA-6.6 MLD. The colours of the frames refer to the corresponding coloured thickness ( c ) and polarimetry ( d ) data points. ( c ) PA-6.6 average thickness as function of the MLD cycles after AFM topography image analysis. The error bars indicate the s.d. from the average thicknesses shown in the inset, which shows the line profiles of all the disks included in the images in b . The line profiles are taken along two orthogonal directions, which are shown as white dashed lines only in the AFM image of the clean sample in b . ( d ) Plot of the inverse of transmitted and reflected light ellipticity λ ε as a function of MLD cycles (black dashed lines are guide for eyes). Surface sensitivities of ~3.1 (transmission) and ~5.4 (reflection) are found combining plots ( c , d ), in excellent agreement with the results presented in Fig. 3 . The horizontal error bars indicate the s.d. from the average thicknesses shown in the inset in ( c ). The vertical error bars indicate the experimental error in the magneto-optical measurements. The insets show the corresponding 1/|Δ ε | spectra for the two measurement geometries (reflection—top-left inset and transmission—bottom-right inset). Full size image Given the surface sensitivity ( S Surf ) values ~3 and ~5.3 of our approach (transmission and reflection geometry, respectively), detection of subnanometre-thick PA-6.6 coverage, namely, a discontinuous monolayer (ML) of PA-6.6 on individual cylindrical Ni nanoantennas is achievable (~1.7 and ~1.0 Å for the two measurement geometries). A ML of PA-6.6 is ~8.5-Å thick [29] , the precision above corresponds, in the case of transmission geometry, to a coverage of less than 0.2 ML, namely a ML covering less than 20% of the nanoantenna-exposed surface. The minimum detectable coverage reduces to 0.1 ML in reflection geometry. Such sub-ML coverage values are equivalent to PA-6.6 volumes of ~1,200 and 800 nm 3 , that is, a remarkable mass sensitivity of ~1.2 and 0.8 ag per disk corresponding to ~3,300 and 2,200 molecules of PA-6.6 per disk (density of amorphous PA-6.6 is 1.05 g cm −3 and its molecular weight is 226 g mol −1 ). Such minimum detectable coverage is based on extrapolation and assumes that the electric near field is uniformly distributed in the vicinity of the Ni nanoantenna surface exposed to the environment, that is, the surface sensitivity is not, or weakly, space-dependent. This condition is fulfilled to a good extent for our nanodisks with a diameter of 100 nm as we verified by the simulations of the near field produced by the excitation of a LPR performed using Lumerical (see Supplementary Fig. 4 ). A raw limit of detection of a few zg per nanoantenna can be achieved considering the submicro-radiant resolution of advanced polarimetry tools. These sensing performances could be further improved by applying the same strategies as employed for noble metal nanoplasmonic systems for label-free detection, such as lifting of the nanostructures from the substrate and exploiting resonant coupling between LPRs to modes with narrow FWHM. In addition, reducing the diameter of the cylindrical Ni nanoantennas would improve the limit of detection, since the surface sensitivity is weakly dependent on the diameter and, consequently, also the ability to detect a ML coverage of 20 and 10% of the nanoantenna-exposed surface, which for smaller nanoantennas corresponds to proportionally smaller volumes of material. So far, the limit of detection of our approach was derived based on the signal-to-noise ratio of the measurements, without any mathematical fit of the data, and compared with those of similar ‘raw’ estimates of sensitivity based on absorption spectrum measurement. This comparison demonstrates the radically improved sensitivity enabled by our nanomagnetoplasmonic approach with respect to plasmon-based sensors. Higher sensitivity and limit of detection values are reported in literature for plasmon-based sensors, which are achieved by application of fitting procedures [30] , [31] . We mention here that the application of fitting procedures of our data confirms the higher sensitivity of our approach as shown in the Supplementary Fig. 5 . Indeed, a mass sensitivity in the sub-zg per nanoantenna, down to a few yg per nanoantenna, can be achieved through the application of fitting procedures opening a pathway to mass sensitivity corresponding to ~10 molecules of PA-6.6 per disk (or, equivalently, of any material having n ~1.5 and a density of ~1 g cm −3 , which is the case of many polymers and biomolecules). Magnetoplasmonic nanoantennas that support magneto-optically induced localized plasmon resonances have been synthesized in order to induce a null condition of the transmitted/reflected light polarization ellipticity at desired wavelengths. The obtained null condition allows for an easily measurable and extremely precise phase-sensitive detection of localized plasmon resonances. Such magnetoplasmonic nanoantennas can be used for optical sensing of local refractive index variations with enhanced sensitivity and unrivalled values for the FoM, even exceeding the theoretically predicted upper limit for sensing based on propagating SPRs. Our approach requires extremely simple and scalable nanostructuring processes and offers a remarkably improved sensitivity performance in a large spectral range. To conclude, we would like to emphasize that the ultrasensitive sensing capabilities of our magnetoplasmonic nanoantennas can be used also in nanoplasmonic biosensing (for instance, cancer serum detection). Ni surfaces are covered by an ultrathin layer of oxidized Ni. Such surfaces can be functionalized with either silanes or even better with Histidin tags (His6) [32] on par with Au surface functionalization with thiolate chemistry, thus informing our selected Ni as the material for our nanoantennas. As an alternative, one could even deposit a thin layer of Au, which will not affect the plasmonic behaviour (even improve it, according to literature), and use conventional thiolate chemistry. In addition to biosensing, there are also many other potential civil and/or military applications that do not require surface functionalization and would enormously benefit from our approach like chemical sensing of toxic materials, explosives and ultra-precise thickness-monitoring applications. Optical and MO measurements The extinction spectra ( I 0 − I t )/ I 0 , where I 0 and I t are the intensities of the incident and transmitted light, respectively, were taken in the wavelength range 420–900 nm. The intensity of the light passing through the substrate without nanostructures on top was taken as the reference I 0 signal. The wavelength dependence of the magneto-optically induced ellipticity change Δ ε of the transmitted or reflected light was measured using MO Faraday (incidence angle 0°) and Kerr (incidence angle 2.5°) effect spectrometers working in polar geometry in the wavelength range 420–950 nm. The incident light beam was linearly polarized with either p- or s-polarization. Δ ε was measured by switching the polarity of a magnetic field H =4 kOe applied normal to the sample plane to activate the MO coupling in the nanoantennas’ constituent material. As shown schematically in Supplementary Fig. 2 , in the polar-Kerr geometry Δ ε was measured at each wavelength with the transmitted beam passing through a photoelastic phase modulator and a polarizer before detection. A lock-in amplifier was used to filter the signal at the modulation frequency in order to retrieve Δ ε (ref. 33 ). Our experimental set-up allows measuring polarization parameters, like ε and Δ ε , with submicro-radiant precision, although in our analysis of the measured spectra we assumed a 5 micro-radians error bar, for the sake of demonstrating that our approach guarantees a high sensitivity even using extremely simple measurement set-ups as that shown in the Supplementary Fig. 6 . It is worth mentioning that Δ ε can be equivalently measured in reflection geometry with the light impinging on either magnetoplasmonic sample surface side ( Fig. 1c ). Measurement of Δ ε with the light beam impinging from the glass bottom surface can be particularly appealing for implementation of our approach in practical devices ( Supplementary Fig. 6 ). Sensing experiments Bulk sensitivity experiments were performed in a microfluidic cell where different liquids, with different refractive index, were injected every time. We used liquids and mixtures whose refractive indexes are well known, namely water (n =1.33), glycerol ( n =1.47) and 50% glycerol volume in water ( n =1.41). For surface sensitivity assessment, MLD of polyamide 6.6 (PA-6.6) was carried out in a commercially available Cambridge Nanotech/Ultratech Savannah system using alternating pulses of adipoyl chloride (AC; Sigma Aldrich) and 1,6-hexamethylenediamine (HD; Sigma Aldrich) with the following pulse/purge/pulse/purge parameters; 0.5 s/30 s/0.5 s/30 s. The AC and HD were heated to 70 and 80 °C, respectively. The reaction chamber was maintained at 85 °C throughout the reaction. Before deposition the samples were treated using 5-min cycles of acetone and isopropanol ultrasonication, and then exposed to Ar plasma at 90 W for 60 s to eliminate residues of organic materials. Coating and cleaning procedures were repeated several times to ensure the reproducibility of the experiment (both polarization and thickness of PA-6.6 deposits). The thickness of the PA-6.6 deposits was monitored via AFM. The AFM measurements were carried out in the same region after each MLD cycles and MOKE measurement step, using an Agilent 5500 AFM microscope with a Si tip operated in tapping mode. The images were analysed using the Gwyddion software package in order to extract the average thickness values of PA-6.6 deposits. Both bulk and surface sensitivity experiments were repeated five times each, giving the same results within the experimental errors reported above. Sample fabrication Bottom-up hole mask colloidal lithography was used to pattern the Ni nanodisks [25] . The following process steps were applied in all presented examples. The substrates used are 10 × 10 × 1 mm 3 pieces of microscope slide glass (VWR International). The glass substrates were first cleaned through 5-min cycles of acetone, isopropanol and water ultrasonication. A poly(methyl methacrylate) (PMMA) film (2 wt % PMMA diluted in anisole, MW=950,000) was spin-coated on a clean surface and followed bysoft baking (170 °C, 10 min on a hot plate). Reactive oxygen plasma treatment (50 W, 5 s, 250 mTorr, Plasma Therm Batchtop RIE 95 m) was applied in order to decrease the polymer film hydrophobicity and avoid spontaneous de-wetting of the surface during subsequent polyelectrolyte and particle deposition steps, which would introduce inhomogenities in the particle distribution. Providing a net charge to the PMMA surface by pipetting a solution containing a positively charged polyelectrolyte on the film (polydiallyldimethylammonium MW 200,000–350,000, Sigma Aldrich, 0.2 wt % in Milli-Q water, Millipore), followed by careful rinsing with de-ionized water in order to remove excess polydiallyldimethylammonium and blow-drying with a N 2 stream. Deposition of a water suspension containing negatively charged polystyrene particles (sulfate latex, Invitrogen, 0.2 wt % in Mili-Q water) and N 2 drying in a similar manner as described above, leaving the PMMA surface covered with uniformly distributed PS-spheres. Evaporation of an oxygen plasma-resistant thin film of Au. Removing the PS spheres using tape stripping (SWT-10 tape, Nitto Scandinavia AB), resulting in a mask with holes arranged in a pattern determined by the self-assembled colloidal particles. Transfer of the hole-mask pattern into the sacrificial layer via an oxygen plasma treatment (50 W, 250 mTorr, Plasma Therm Batchtop RIE 95 m), which effectively removes all PMMA situated underneath the holes in the film, leaving the surface covered with a thin-film mask supported on a perforated, undercut polymer film. Ni deposition is carried out by e-beam-assisted evaporation (AVACHVC600). Lift off was carried out using acetone at room temperature or 50 °C for 5–10 min. The filling factor (surface covered by Ni nanoantennas normalized to area of the sample surface) can be varied between 5 and 30% in a controlled manner. The filling factor of the samples utilized in our experiments can be estimated to be around 15%. How to cite this article: Maccaferri, N. et al . Ultrasensitive and label-free molecular-level detection enabled by light phase control in magnetoplasmonic nanoantennas. Nat. Commun. 6:6150 doi: 10.1038/ncomms7150 (2015).